Chemical synthesis of perfectly isotactic and high melting bacterial poly(3-hydroxybutyrate) from bio-sourced racemic cyclic diolide Bacterial poly(3-hydroxybutyrate) (P3HB) is a perfectly isotactic, crystalline material possessing properties suitable for substituting petroleum plastics, but high costs and low volumes of its production are impractical for commodity applications. The chemical synthesis of P3HB via ring-opening polymerization (ROP) of racemic β -butyrolactone has attracted intensive efforts since the 1960s, but not yet produced P3HB with high isotacticity and molecular weight. Here, we report a route utilizing racemic cyclic diolide ( rac -DL) derived from bio-sourced succinate. With stereoselective racemic catalysts, the ROP of rac -DL under ambient conditions produces rapidly P3HB with perfect isotacticity ([ mm ] > 99%), high melting temperature ( T m = 171 °C), and high molecular weight ( M n = 1.54 × 10 5 g mol −1 , Đ = 1.01). With enantiomeric catalysts, kinetic resolution polymerizations of rac -DL automatically stops at 50% conversion and yields enantiopure ( R,R )-DL and ( S,S )-DL with >99% e.e . and the corresponding poly[( S )-3HB] and poly[( R )-3HB] with high T m = 175 °C. Poly(hydroxyalkanoate)s (PHAs) [1] , [2] , [3] , [4] , [5] , [6] , [7] , [8] , [9] , [10] , [11] , [12] , naturally produced by bacteria and other living microorganisms from biorenewable resources such as carbohydrates and fats, are an important class of commercially implemented aliphatic polyesters as biodegradable and/or biocompatible materials for biomedical, pharmaceutical, and packaging applications [13] , [14] , [15] , [16] , [17] , [18] , [19] , [20] . The most prominent, thus most extensively studied, PHA is poly(3-hydroxybutyrate) (P3HB), in which bacterial poly[( R )-3-hydroxybutyrate], P[( R )-3HB], is a perfectly stereoregular, pure isotactic crystalline thermoplastic material [1] , [2] , [3] , [4] , [5] , [6] , [7] , [8] , [9] , [10] , [11] , [12] . Thanks to its comparable thermal and mechanical properties to those of high-performance isotactic polypropylene ( it -PP), highly isotactic P3HB is being considered as an attractive biodegradable alternative to petroleum-based plastics, especially it -PP. However, high current production costs and limited production volumes of bacterial/microbial PHAs, including P3HB, render them impractical in many applications in areas such as biorenewable and biodegradable green commodity thermoplastics. The chemical synthesis via ring-opening polymerization (ROP) of cyclic esters (lactones or lactides), a process typically catalyzed by a metal-based or organic catalyst, offers an alternative route to such technologically important biodegradable aliphatic polyesters [21] , [22] , [23] , [24] , [25] , [26] , [27] , [28] , which is often advantageous, thanks to its fast kinetics of the polymerization, scalability of the polymer production, and tunability of catalysts and co-monomers. In this context, the ROP of β -butyrolactone ( β -BL) has been developed for the chemical synthesis of P3HB [29] , [30] , [31] , [32] , [33] , while the ROP of γ -butyrolactone ( γ -BL) for the chemical synthesis of poly(4-hydroxybutyrate) (P4HB) [34] , [35] has also been realized recently [36] . In the case of the ROP of β -BL, the cost-effective chemical synthesis of P3HB calls for the use of the racemic monomer, rac - β -BL, rather than the more expensive enantiopure ( R )- β -BL, which requires a stereoselective ROP process to render the formation of isotactic P3HB. However, despite extensive research efforts since the 1960s, the chemical synthesis of P3HB with isotacticity P m (defined as the probability of meso linkages between monomer units) >0.85 from the ROP of rac - β -BL has proven elusive. For example, the ROP of rac - β -BL by alkyl aluminoxanes produced a mixture of iso-enriched P3HB products as a whole ( P m = 0.62), which were fractionated into atactic and isotactic fractions with the highest P m of 0.85 reported for the acetone-insoluble fraction [37] , [38] , [39] . A chiral initiator system consisting of ZnEt 2 /( R )(−)-3,3-dimethyl-1,2-butanediol also yielded a mixture of P3HB products that were fractionated in methanol into soluble atactic and insoluble (~25%) isotactic ( P m ~ 0.80) fractions [40] , and a chiral Co(salen)/Et 3 Al complex afforded P3HB of low crystallinity (no tacticity data) [41] . A discrete β -diiminate zinc alkoxide initiator promoted a controlled ROP of rac - β -BL with high polymerization rates, but the resulting P3HB is atactic [42] . Cr(III) salophen complexes converted rac - β -BL into iso-enriched P3HB with P m = 0.66, medium number-average molecular weight ( M n = 4.81 × 10 4 g mol −1 ), high dispersity ( Đ = 5.2), and modest melting-transition temperature ( T m = 116, 142 °C) [43] . Lanthanide (La, Nd) borohydrides supported on silica polymerized rac - β -BL into P3HB with P m = 0.85 and M n = 1.15 × 10 4 g mol −1 [44] . It is worth noting that syndiotactic P3HB materials from being modestly syndiotactic ( P r ~ 0.70) [45] , [46] to highly syndiotactic ( P r up to 0.95) [47] , [48] , [49] , have been achieved through the ROP of rac - β -BL using alkyltinoxides and discrete yttrium complexes [50] supported by tetradentate, dianionic alkoxy-amino-bis(phenolate) [ O − , N , O , O − ] ligands, respectively. This Y catalyst system has also been utilized for the ROP of functional β -lactones, such as 4-allyloxymethylene- β -propiolactone, to afford either highly isotactic ( P m = 0.93, M n = 9.20 × 10 3 g mol −1 , Đ = 1.46) or syndiotactic ( P r = 0.91) polymer, depending on the substituents on the ligand [51] . In the context of creating a synthetic equivalent of bacterial P3HB, both high isotacticity ( P m > 0.95) and molecular weight ( M n > 10 5 g mol −1 ) are typically required for practical use. It is informative to point out that the ingenious utilization of a cyclic dimer of l -lactic acid ( l -LA) rendered the commercial production of high-molecular-weight, highly isotactic polylactide (PLA) [52] , but the efforts in attempting the chemical synthesis of high-molecular-weight, highly isotactic P3HB have so far been strictly limited to the use of the cyclic monomer of 3-hydroxybutyric acid (3HB), namely β -BL. β -Lactones are known to be carcinogenic (alkylating DNA) [53] , and the competing ring-opening mechanisms (O-acyl vs. O-alkyl cleavage) were reported for the ROP of such highly strained monomers [54] , [55] , [56] . As the current approach via the ROP of rac - β -BL has yet so far produced P3HB with high molecular weight and high isotacticity (vide supra), we formulated the following three working hypotheses to address this long-standing challenge. First, by analogy of the PLA production, the chemical synthesis of P3HB could utilize a cyclic dimer of 3HB, namely eight-membered cyclic diolide (DL, Fig. 1 ), which is benign and can be readily derived from bio-sourced dimethyl succinate [57] . Worth noting here is that the enantiopure cyclic trimer of ( R )-3HB, obtained in ~50% yield from the depolymerization of bacterial P[( R )-3HB] [58] , was attempted to polymerize back to P3HB but only low molecular weight ( M n ~ 5000 g mol −1 ) oligomers were obtained [59] , [60] . Second, as DL possesses two stereogenic centers, the ROP of its rac and meso diastereomers could lead to various stereoregular (isotactic, syndiotactic, stereoblock, etc.) P3HB materials, depending on the stereoselectivity of the catalyzed ROP process. Third, considering significantly increased sterics present in DL relative to β -BL, we should anticipate a higher degree of stereochemical control in the catalyzed ROP of DL, thereby potentially generating highly stereoregular P3HB materials. Fig. 1 Chemical synthesis routes to P3HB. a Classical route via the ROP of rac - β -BL to iso-enriched P3HB. b The new route via the ROP of rac -DL to perfectly isotactic P3HB. ( P m is the probability of meso linkages between HB units, and mm is isotactic triad made up of two adjacent meso diads) Full size image Guided by the above three hypotheses, we have investigated this proposed DL route to P3HB and hereby disclose our discovery that the catalyzed ROP of rac -DL (Fig. 1 ) enables the highly efficient synthesis of P3HB with perfect isotacticity, high crystallinity, high melting temperature, and high molecular weight. Stereoselective ROP of rac -DL Pure rac -DL can be synthesized in a multi-gram scale from bio-sourced dimethyl succinate (Supplementary Figs. 2 – 6 ; see Supplementary Information for details.). At the outset, the ROP of rac -DL was screened with La[N(SiMe 3 ) 2 ] 3 ( 1 ), a lanthanum complex that has been shown to be an effective catalyst for the ring-opening (co)polymerization of γ -BL and α -methylene- γ -butyrolactone (MBL) [36] , [61] , [62] . 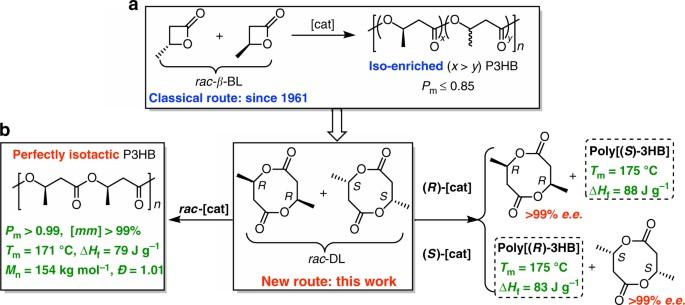Fig. 1 Chemical synthesis routes to P3HB.aClassical route via the ROP ofrac-β-BL to iso-enriched P3HB.bThe new route via the ROP ofrac-DL to perfectly isotactic P3HB. (Pmis the probability of meso linkages between HB units, andmmis isotactic triad made up of two adjacentmesodiads) In combination with an alcohol initiator, the 1 / x BnOH ( x = 2, 3, BnOH = benzyl alcohol) system was effective for the ROP of rac -DL (20 equiv) in dichloromethane (DCM) at room temperature (RT), achieving 100% conversion ( x = 2) in 4 h or 98% ( x = 3) conversion in 8 h, but the resulting P3HB exhibited a low molecular weight ( M n = 2.43 × 10 3 g mol −1 and Đ = 1.09 for x = 3, Supplementary Table 1 ). Furthermore, both 1 H and 13 C NMR spectra (Supplementary Figs. 32 , 33 ) showed the formation of an iso-biased amorphous material ( P m = 0.74, x = 2; P m = 0.70, x = 3), which was confirmed by observation of only glass-transition temperature ( T g ) on its differential scanning calorimetry (DSC) curves (Supplementary Fig. 34 ). Next, we turned to a “privileged class of catalysts” for the ROP of cyclic esters [21] , discrete yttrium amido complexes 2 ( a , R = t Bu; b , R = CMe 2 Ph) and alkyl complex 3 supported by the tetradentate [ O − , N , O , O − ] ligand (Fig. 2 ), which were previously shown to be superior catalysts for the ROP of γ -BL and MBL [36] , [61] , [62] as well as highly active catalysts for the syndiospecific ROP of rac - β -BL [47] , [48] , [49] . With a high precatalyst loading of 5 mol% and in combination with 1 equiv of BnOH initiator that undergoes instantaneous alcoholysis of the yttrium complex to generate the corresponding yttrium alkoxide catalyst [47] , [48] , [49] , [50] , all three yttrium complexes were active for the ROP of rac -DL, with yttrium alkyl 3 being the most active but still rather sluggish (76% conversion after 32 h). Moreover, these catalysts incorporating the tripodal alkoxy-amino-bis(phenolate) ligand afforded only low-molecular-weight ( M n = 2.70 × 10 3 g mol −1 and Đ = 1.08 for catalyst 3 ), iso-biased amorphous material ( P m = 0.76, Supplementary Table 1 , Supplementary Figs. 35 , 36 ). For catalysts 2 , only low conversions were achieved even after 48 h (44% by 2a ; 17% by 2b ), and the P3HB products were not isolated but the estimated P m values by in situ NMR spectra were similar to that by catalyst 3 . Fig. 2 Chemical structures of the catalysts. Structures of catalysts employed in this study for the ROP of rac -DL and the isotacticity of the resulting P3HB materials they produced. ( P m is the probability of meso linkages between HB units, and mm is isotactic triad made up of two adjacent meso diads) Full size image Considering the steric hindrance of rac -DL monomer with the eight-membered-ring framework and the low activity and isoselectivity of also sterically encumbered catalysts 1 – 3 screened, we arrived at sterically more open yttrium racemic salen complexes 4a – e (Fig. 2 ). Yttrium silylamido complexes 4a – d supported by N,N′ -bis(salicylidene)cyclohexanediimine (salcy) ligands and complex 4e supported by the analogous salph ligand were readily synthesized in good yields (58–83%, see Supplementary Information for details, Supplementary Figs. 13 – 22 ) according to the procedures established for the synthesis of known complex 4a [63] , [64] and known salen ligands (Supplementary Figs. 7 – 13 ) [65] , [66] , [67] , [68] , [69] , [70] , [71] . Complex 4a with the classic salen ligand bearing the 3, 5-di- tert -butyl substituents was first examined for its activity and stereoselectivity towards the ROP of rac -DL. Excitingly, this complex, when combined with 1 equiv of BnOH initiator, rapidly polymerized 20–200 equiv of rac -DL to completion within 20 min at RT. The molecular weight of the resulting P3HB increased from low M n = 4.77 × 10 3 g mol −1 ( Đ = 1.17) to medium M n = 3.20 × 10 4 g mol −1 ( Đ = 1.03) with increasing the [ rac -DL]/[ 4a ] ratio from 20/1 to 200/1, and the calculated initiation efficiency ranged from 74 to 108% (runs 1–4, Table 1 ), all indicating a controlled polymerization. More importantly, complex 4a now yielded isotactic P3HB with P m ~ 0.91–0.94 and isotactic [ mm ] triad ~ 87–89% based on 1 H and 13 C NMR analysis (Fig. 3 ). Accordingly, the resulting P3HB material became crystalline, exhibiting a T m ~ 136–146 °C, depending on the polymer molecular weight (runs 1–4, Table 1 ). Replacing the initiator BnOH with i PrOH lowered the polymerization activity by threefold, now requiring 60 min to achieve complete monomer (200 equiv) conversion. Furthermore, the molecular weight ( M n = 6.07 × 10 4 g mol −1 ) of the resulting P3HB was considerably higher than the theoretical value, thus giving rise to a low initiation efficiency of only 57%, although the P3HB tacticity remained the same. Other alcohols such as Ph 2 CHCH 2 OH were also found less effective than BnOH. Therefore, all the subsequent polymerization studies with other yttrium complexes ( 4b – e ) employed exclusively BnOH as the more effective initiator. Table 1 Results of rac -DL polymerization by yttrium catalysts 4a–e and BnOH initiator Full size table Fig. 3 Stereomicrostructures (tacticities) of P3HB. a 1 H NMR spectra (CDCl 3 ) in the methylene region. b 13 C NMR spectra (CDCl 3 ) in the carbonyl, methylene, and methyl regions. P3HB produced by (1a–b) [ rac -DL]/[ 4a ] = 200/1; (2a–b) [ rac -DL]/[ 4b ] = 200/1; (3a–b) [ rac -DL]/[ 4c ] = 200/1; (4a–b) [ rac -DL]/[ 4d ] = 200/1; (5a–b) [ rac -DL]/[ 4e ] = 200/1; and (6a–b) comparative example of [ rac - β -BL]/[ 4d ] = 100/1 Full size image The above exciting results brought about by yttrium salen complex 4a prompted us to investigate possible effects of the salen ligand framework’s electronics, sterics, and geometry of the backbone diimine linker on the rac -DL polymerization activity and stereoselectivity. In the context of electronic effects, electron withdrawing substituents (e.g., F) introduced to the 5-positions of the salicylidene framework were found to generate a more redox stable and active (salcy)Co(III) catalyst for the copolymerization of epoxide and anhydride monomer pairs [65] . In the present polymerization of rac -DL by (salcy)yttrium catalyst 4b with the F groups substituted at the 5-positions of the salcy ligand, only the isotacticity of the resulting P3HB was improved slightly to now P m = 0.95 and T m = 147 °C (runs 5 and 6, Table 1 ), as compared with the parent tert -butyl substituted catalyst 4a . Turning to the steric perturbation of the catalyst, the more bulky cumyl-substituted complex 4c produced isotactic P3HB with a noticeably higher isotactic [ mm ] triad of 94% (Fig. 3 ) and T m of 156 °C (run 8, Table 1 ), relative to the [ mm ] of 89% and T m of 146 °C for the P3HB produced by catalyst 4a under identical conditions (run 4 vs. 8, Table 1 ). These results showed much more pronounced effects of the ligand sterics than electronics on the polymerization stereoselectivity. Hence, the even more bulky trityl (Ph 3 C) groups were substituted at the 3-positions of the salcy ligand framework to generate catalyst racemic 4d . Remarkably, catalyst 4d produced essentially stereo-perfect, pure isotactic P3HB with P m > 0.99 and [ mm ] > 99% (run 10, Table 1 ), while maintaining high polymerization activity (100% monomer conversion in 20 min). Consistent with this NMR-derived stereo-microstructure (Fig. 3 ), the resulting crystalline isotactic P3HB exhibited a high T m of 164 °C. Lastly, to probe the possible effects of the geometry of the backbone diimine linker, we examined the performance of the salph-based complex 4e for the rac -DL polymerization and found that this catalyst afforded P3HB with a considerably lower isotacticity ( P m ~ 0.88–0.89, [ mm ] = 79%, runs 14 and 15), as compared with the salcy-based analogue complex 4a under identical conditions ( P m ~ 0.93–0.94, [ mm ] = 89%, runs 3 and 4). It is worth noting here that the high stereoselectivity of catalysts 4 observed for the ROP of rac -DL does not apply to the ROP of rac - β -BL; for example, the ROP of rac - β -BL by the best catalyst of the series, 4d , was not only sluggish (even with a high catalyst loading of  1.0 mol% the reaction required 8 h to achieve 96% monomer conversion) but also non-stereoselective, producing atactic P3HB (Fig. 3 , Supplementary Fig. 40 ). These results further highlight the importance of the steric interplay and matching between the catalyst and monomer structures to achieve a highly stereoselective ROP of such racemic lactone and diolide monomers. Having identified catalyst 4d being the best catalyst of this series, we further examined the ability of this catalyst to control the molecular weight so that practically useful high-molecular-weight isotactic P3HB with M n > 10 5 g mol −1 could be synthesized. To this end, we varied the [ rac -DL]/[ 4d ] feed ratio from 100/1 to 1200/1 and found that the molecular weight of the resulting P3HB increased linearly ( R 2 = 0.997, Fig. 4 ) from medium M n = 2.01 × 10 4 g mol −1 ( Đ = 1.07) to high M n = 1.54 × 10 5 g mol −1 ( Đ = 1.01), while all the Đ values remained low in a narrow range from 1.01 to 1.07 (runs 9–13, Table 1 ). These observations, coupled with the calculated high initiation efficiencies of >86% for all the polymerization runs by catalyst 4d , pointed to a well-controlled ROP of rac -DL. Fig. 4 Degree of control over the molecular weight and dispersity in the ROP of rac -DL. Plots of M n and Đ values of isotactic P3HB produced by racemic catalyst 4d at varied [ rac -DL]/[ rac - 4d ] ratios. The runs at 800/1 and 1200/1 ratios under the same conditions (0.8 mL DCM, 60 min) did not achieve quantitative conversions; thus, the ratios used for the plot were adjusted by their conversions (98% and 74%, respectively) Full size image Thermal properties DSC curves of the isotactic P3HB materials produced by the ROP of rac -DL with catalysts 4a – 4d under identical conditions ([ rac -DL]/[ 4 ] = 200/1, DCM, RT, 20 min, 100% conversion) are compared in Fig. 5 . Consistent with the gradual increase of the isotacticity of P3HB on going from 4a to 4d , the T m value was observed to increase from 146 ( 4a ) to 147 ( 4b ), 156 ( 4c ), and 164 °C ( 4d ). Noteworthy also is the steadily enhanced heat of fusion (∆ H f ) from 4a to 4d : 40.9, 47.0, 56.5, and 79.3 J g −1 , which corresponds to an increase in the P3HB crystallinity from 28 to 32, 39, and 54%, relative to the estimated ∆ H f 0 value (146 J g −1 ) for an infinite crystal of 100% crystalline P3HB (Supplementary Note 1 ) [72] . Furthermore, the T m value of the perfectly isotactic P3HB produced by catalyst 4d depends somewhat on the polymer M n : when M n was enhanced from 2.01 × 10 4 to 3.74 × 10 4 , 6.43 × 10 4 , 1.19 × 10 5 , and 1.54 × 10 5 g mol −1 (runs 9–13, Table 1 ), T m increased accordingly from 161 to 164, 169, 170, and 171 °C. These are perfectly isotactic, highly crystalline materials, with high ∆ H f values of ~ 80 J g −1 (Fig. 5 , Supplementary Fig. 40 ). Fig. 5 Thermal properties of P3HB derived from the ROP of rac -DL. a [ rac -DL]/[ 4a ] = 200/1 (∆ H f = 40.9 J g −1 ). b [ rac -DL]/[ 4b ] = 200/1 (∆ H f = 47.0 J g −1 ). c [ rac -DL]/[ 4c ] = 200/1 (∆ H f = 56.5 J g −1 ). d [ rac -DL]/[ 4d ] = 200/1 (∆ H f = 79.3 J g −1 ). e [ rac -DL]/[ 4d ] = 400/1 (∆ H f = 80.4 J g −1 ). f [ rac -DL]/[ 4d ] = 1200/1 (∆ H f = 78.6 J g −1 ). Crystallization temperature ( T c ) and melting-transition temperature ( T m ) taken from the cooling and second heating scans, respectively Full size image Thermal degradation profiles of the selected isotactic P3HB samples derived from the ROP of rac -DL by racemic  catalysts 4a and 4d were examined by thermal gravimetric analysis (TGA). As can be seen from the TGA and derivative thermogravimetry (DTG) curves (Fig. 6 ), the P3HB produced by 4a ( M n = 3.20 × 10 4 g mol −1 , Đ = 1.03, [ mm ] = 89%) exhibited a decomposition temperature ( T d ) (defined by the temperature of 5% weight loss in the TGA curve) of 234 °C and a maximum rate decomposition temperature ( T max ) of 274 °C, which put the T d ~ 90 °C above its T m , proving a window for melt processing. A P3HB sample produced by 4d with a similar M n (3.74 × 10 4 g mol −1 ) but a much higher isotacticity of [ mm ] > 99% exhibited a somewhat higher T d of 239 °C and T max of 281 °C (Supplementary Fig. 41 ). Keeping the tacticity the same ([ mm ] > 99%) while increasing the molecular weight to M n = 1.19 × 10 5 g mol −1 enhanced the T d only slightly to 241 °C (Fig. 6 ). Fig. 6 Thermal stability of P3HB derived from the ROP of rac -DL. a TGA and DTG of P3HB produced by catalyst 4a , M n = 3.20 × 10 4 g mol −1 , Đ = 1.03, [ mm ] = 89%. b TGA and DTG of P3HB produced by catalyst 4d , M n = 1.19 × 10 5 g mol −1 , Đ = 1.03, [ mm ] > 99% Full size image Kinetic resolution and mechanistic considerations The above results demonstrated that the polymerization of rac -DL by rac - 4d produced P3HB with essentially perfect isotacticity. However, these exciting results also brought about three important fundamental questions: (1) Can enantiomeric catalysts ( R,R )- 4d and ( S,S )- 4d kinetically resolve racemic monomer rac -DL? (2) What is the stereocontrol mechanism—enantiomorphic-site control or chain-end control? (3) What is the isotactic polymer stereomicrostructure—1:1 mixture of poly[( R,R )-DL] and poly[( S,S )-DL], stereoblock of poly( rac -DL), or tapered block copolymer poly[( R,R )-DL]- co -[( S,S )-DL]? To address these questions, the corresponding enantiomeric catalysts ( R,R )- 4d and ( S,S )- 4d have been successfully synthesized and subsequently employed to perform kinetic resolution polymerization of rac -DL with both enantiomeric catalysts (See Supplementary Information for details, Supplementary Figs. 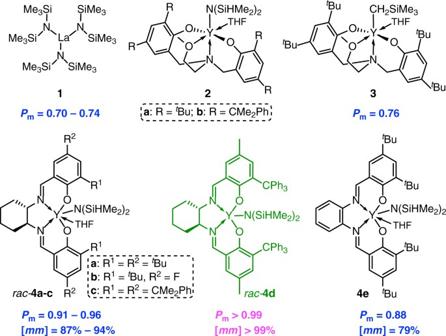Fig. 2 Chemical structures of the catalysts. Structures of catalysts employed in this study for the ROP ofrac-DL and the isotacticity of the resulting P3HB materials they produced. (Pmis the probability of meso linkages between HB units, andmmis isotactic triad made up of two adjacentmesodiads) 23 – 29 ), the results of which are summarized in Table 2 . In sharp contrast to the polymerization by rac - 4d with a [ rac -DL]/[ rac - 4d ] ratio of 400 or 800 that achieved a quantitative monomer conversion after 20 min, the same polymerization by ( R,R )- 4d or ( S,S )- 4d achieved a conversion of ~50% (runs 1–2 and 4–5, Table 2 ), after which no further monomer conversion can be achieved, even after extended times (6 h), indicative of exclusive catalyst site selectivity for the ROP of one particular enantiomer of the monomer. Characterizations of the ~50% unreacted, pure monomer showed to exhibit identical NMR spectra to that of rac -DL (Supplementary Fig. 42 ); the specific rotation of the unreacted monomer produced by ( R,R )- 4d was measured to be from −94.8° to −94.5° (runs 1–2, Table 2 ), which agrees well with the reported value of ( R,R )-DL [57] , while the specific rotation of the unreacted monomer by ( S,S )- 4d was from +93.7 to +94.6 (runs 4–5, Table 2 ), which is assigned to be ( S,S )-DL accordingly. The enantiomeric excess ( e.e .) of the unreacted monomer was determined by chiral HPLC coupled with a Chiralcel OD-H column to be >99% e.e . (Supplementary Figs. 55 , 56 and 58 , 59 ) for all the runs with conversion at ~50% (runs 1–2 and 4–5, Table 2 ). It is noted here that the [ rac -DL]/[ 4d ] = 1600 runs achieved 43–44% conversion after 60 min (runs 3 and 6); accordingly, the e.e .’s of the unreacted monomer was only 80–85%, respectively (Supplementary Figs. 57 and 60 ). Overall, these results indicate that ( R,R )- 4d exhibits exclusive selectivity for the ROP of ( S,S )-DL, while ( S,S )- 4d polymerizes ( R,R )-DL exclusively. Based on the quantitative e.e .’s (>99%) for the optically resolved, unreacted monomer, the stereoselectivity factor s for both enantiomeric catalysts was calculated to be >10 3 . These profound results also indicated an enantiomorphic-site control mechanism for the stereoselective ROP process. 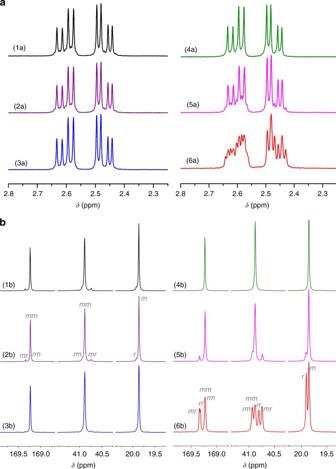Fig. 3 Stereomicrostructures (tacticities) of P3HB.a1H NMR spectra (CDCl3) in the methylene region.b13C NMR spectra (CDCl3) in the carbonyl, methylene, and methyl regions. P3HB produced by (1a–b) [rac-DL]/[4a] = 200/1; (2a–b) [rac-DL]/[4b] = 200/1; (3a–b) [rac-DL]/[4c] = 200/1; (4a–b) [rac-DL]/[4d] = 200/1; (5a–b) [rac-DL]/[4e] = 200/1; and (6a–b) comparative example of [rac-β-BL]/[4d] = 100/1 Table 2 Results of rac -DL polymerization by yttrium catalysts ( R,R )- and ( S,S )- 4d /BnOH Full size table This essentially perfect stereoselectivity enabled the synthesis of enantiomeric poly[( R,R )-DL] and poly[( S,S )-DL] using ( S,S )- 4d and ( R,R )- 4d , respectively. The T m values (Table 2 , Supplementary Fig. 43 ) of these enantiopure polymers are somewhat higher (by 3–5 °C) than those of isotactic poly( rac -DL) with similar molecular weights, prepared by rac - 4d , and also higher (by 5–7 °C) than that of 1:1 mixture of poly[( R,R )-DL] and poly[( S,S )-DL] (Supplementary Figs. 44 – 46 ), indicating no stereocomplexation between two enantiomeric P3HB chains. These enantiopure polymers also exhibit high ∆ H f values in the range of 79–88 J g −1 , comparable to that of natural poly[( R )-3HB]. The highest T m of 175 °C was achieved by the enantiomeric polymers with M n = 113–118 kg mol −1 (runs 3 and 6, Table 2 ), which, along with the heat of fusion value, is essentially identical to that of the commercial natural poly[( R )-3HB] (Fig. 7 ). Fig. 7 DSC curves of poly[( R )-3HB] materials. a Produced via chemical ROP of rac -DL by ( S,S )-[ 4d ]. b Commercial natural poly[( R )-3-hydroxybutyric acid] purchased from Sigma-Aldrich. T c and T m values taken from the cooling and second heating scans, respectively Full size image To gain further insight into the stereomicrostructure of the highly isotactic P3HB produced by rac - 4d , the polymers produced at different times and [ rac -DL]/[ rac - 4d ] ratios were analyzed by matrix-assisted laser desorption/ionization time-of-flight mass spectroscopy (MALDI-TOF MS). When a low ratio of 20/1 was used with a longer reaction time (20 min), the mass spectra showed the pronounced transesterification side reaction, as evidenced by the appearances of molecular ion peaks with the spacing between the neighboring peaks being that of the half molar mass of the repeat unit, DL ( m / z = 172.07) (Supplementary Fig. 47 ), which also resulted in a higher dispersity ( Ð = 1.20) and lower isotacticity ( P m = 0.96). Under these conditions, the microstructure of the resultant isotactic P3HB is a stereoblock polymer, poly[( R )-3HB]- b -poly[( S )-3HB], as a result of transesterification after the reaction reached full conversion (Supplementary Fig. 50 ). Consistent with this reasoning, when the polymerization was quenched after 30 s (at which time the full conversion was also achieved), the dispersity of the resulting polymer decreased to Ð = 1.09, and its mass spectrum displayed nearly exclusive molecular ion peaks with the spacing between the neighboring peaks being that of rac -DL, with just minor peaks with extremely low intensity for the odd 3-HB units (Supplementary Fig. 51 ). These results indicate that the transesterification side reaction occurred when the reaction reached full conversion and thus can be essentially shut down by reducing the polymerization time. In this case, the resulting polymer is predominately a mixture of poly[( R )-3HB] and poly[( S )-3HB], with only a trace amount of stereoblock polymer, poly[( R )-3HB]- b -poly[( S )-3HB]. Obviously, the transesterification side reaction can also be shut down by reducing the catalyst amount in feed with the same reaction time, giving the polymers with very low dispersity indices ( Ð = 1.01–1.03) at higher [ rac -DL]/[ rac - 4d ] feeding ratios. Furthermore, this transesterification side reaction can be shut down by the use of enantiomeric pure catalysts (Supplementary Figs. 52 , 53 ). Overall, the polymerization of rac -DL by rac - 4d , when stopped at full conversion (i.e., no transesterification side reactions), produces a mixture of poly[( R )-3HB] and poly[( S )-3HB] (Fig. 8 ), due to its exclusive ( R,R )- 4d /( S,S )-DL and ( S,S )- 4d /( R,R )-DL catalyst/monomer selectivity as demonstrated by the kinetic resolution results. Fig. 8 Proposed mechanism. Chemical scheme of the proposed catalyst-site controlled coordination-insertion mechanism for the ROP of rac -DL by rac - 4d Full size image The approach via the ROP of the bio-sourced rac -DL has successfully addressed the 50+-year challenge in the chemical synthesis of bacterial P3HB. This success was enabled by the specifically designed stereoselective molecular catalyst and its steric interplay with the monomer structure, thereby producing the desired P3HB material with perfect isotacticity ([ mm ] > 99%), high crystallinity, and melting temperature ( T m = 171 °C), as well as high molecular weight and low dispersity ( M n = 154 kg mol −1 , Đ = 1.01). This novel ROP of rac -DL also exhibits a high polymerization rate and efficiency. The resulting highly isotactic P3HB by rac - 4d is shown to be the mixture of poly[( R )-3HB] and poly[( S )-3HB] when the polymerization is stopped at full conversion. 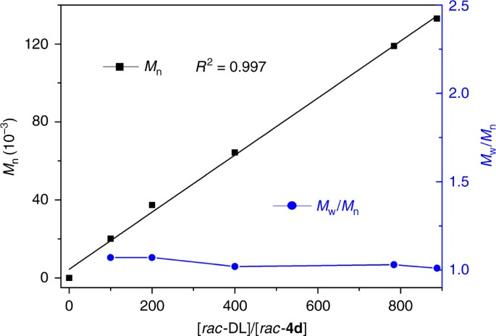Fig. 4 Degree of control over the molecular weight and dispersity in the ROP ofrac-DL. Plots ofMnandĐvalues of isotactic P3HB produced by racemic catalyst4dat varied [rac-DL]/[rac-4d] ratios. The runs at 800/1 and 1200/1 ratios under the same conditions (0.8 mL DCM, 60 min) did not achieve quantitative conversions; thus, the ratios used for the plot were adjusted by their conversions (98% and 74%, respectively) Thanks to the exclusive ( R,R )- 4d /( S,S )-DL and ( S,S )- 4d /( R,R )-DL catalyst/monomer selectivity, kinetic resolution polymerization of rac -DL with enantiomeric catalysts automatically ceases at 50% conversion and yields enantiopure ( R,R )-DL and ( S,S )-DL with >99% e.e . and the corresponding poly[( S )-3HB] and poly[( R )-3HB] with high T m = 175 °C and crystallinity, which is essentially identical to that of the commercial natural poly[( R )-3HB]. The tunability of the catalyst structure allows a rapid entry to P3HB materials with various tacticities (thus tunable thermal and mechanical properties) and predicted molecular weights with low dispersity indices (vs. a typical Đ value of ~2.0 for bacterial P3HB). In addition, the molecular catalysts should allow copolymerization of rac -DL with other monomers to produce 3HB-based copolymers. Altogether, this ROP of DL represents a paradigm shift in the chemical synthesis of P3HB and opens up a plethora of opportunities for discovering new catalysts, materials, and processes in the ROP of rac -DL and other diastereomers of 3HB cyclic dimers or trimers, and so on. Materials and instruments All syntheses and manipulations of air- and moisture-sensitive chemicals and materials were carried out in flamed Schlenk-type glassware on a dual-manifold Schlenk line or in an inert gas (Ar or N 2 )-filled glovebox. NMR-scale reactions were conducted in Teflon-valve-sealed J. Young-type NMR tubes. HPLC-grade organic solvents were first sparged extensively with nitrogen during filling 20 L solvent reservoirs and then dried by passage through activated alumina (for DCM) followed by passage through Q-5 supported copper catalyst (for toluene and hexanes) stainless steel columns. Benzene- d 6 was dried over sodium/potassium alloy and filtered, whereas CD 2 Cl 2 and CDCl 3 were dried over CaH 2 , vacuum-distilled and stored over activated Davison 4 Å molecular sieves. HPLC chromatograms were obtained on an Agilent 1100 series system using a Chiralcel OD-H column with hexanes/isopropanol (80/20) as the eluent at a flow rate of 1.0 mL min −1 . Optical rotations were measured with an Autopol-III automatic polarimeter. NMR spectra were recorded on a Varian Inova or Bruker AV-III 400 MHz spectrometer (400 MHz, 1 H; 100 MHz, 13 C). Chemical shifts for 1 H and 13 C spectra were referenced to internal solvent resonances and are reported as parts per million relative to SiMe 4 . Elemental analyses were performed by Robertson Microlit Laboratories, Madison, NJ. Tri[ N , N -bis(trimethylsilyl)amide] lanthanum(III) La[N(SiMe 3 ) 2 ] 3 ( 1 ), yttrium chloride YCl 3 , and (trimethylsilyl)methyllithium (SiMe 3 ) 2 CH 2 Li solution in pentane were purchased from Sigma-Aldrich Chemical Co. and used as received. 2,2-Diphenylethanol was purchased from Aldrich Chemical Co., which were purified by sublimation twice. Isopropanol and benzyl alcohol were purchased from Fisher Scientific Co. and Alfa Aesar Chemical Co., respectively, which were purified by distillation over CaH 2 and stored over activated Davison 4 Å molecular sieves. Dimethyl succinate, sodium methoxide, and 3-chloroperoxybenzoic acid (mCPBA, 70–75%) were purchased from Fisher Scientific Co. and used as received. Iodomethane was purchased from Alfa Aesar Chemical Co. and used as received. General polymerization procedures Polymerizations were performed in 5.5 mL glass reactors inside the inert glovebox at RT. The reactor was charged with a predetermined amount of catalyst and/or initiator and solvent (as specified in the polymerization tables) in a glovebox. The mixture was stirred at RT for 10 min, and the polymerization was initiated by rapid addition of rac -DL solution. 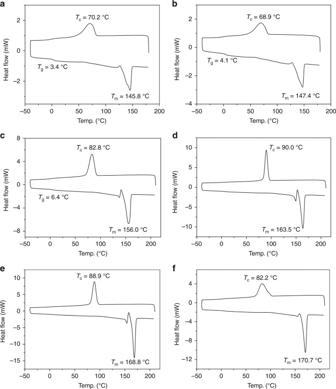Fig. 5 Thermal properties of P3HB derived from the ROP ofrac-DL.a[rac-DL]/[4a] = 200/1 (∆Hf= 40.9 J g−1).b[rac-DL]/[4b] = 200/1 (∆Hf= 47.0 J g−1).c[rac-DL]/[4c] = 200/1 (∆Hf= 56.5 J g−1).d[rac-DL]/[4d] = 200/1 (∆Hf= 79.3 J g−1).e[rac-DL]/[4d] = 400/1 (∆Hf= 80.4 J g−1).f[rac-DL]/[4d] = 1200/1 (∆Hf= 78.6 J g−1). Crystallization temperature (Tc) and melting-transition temperature (Tm) taken from the cooling and second heating scans, respectively After a desired time period, the polymerization was immediately quenched by addition of 0.5 mL of benzoic acid/chloroform (10 mg mL −1 ) and a 0.02 mL of aliquot was taken from the reaction mixture and prepared for 1 H NMR analysis to obtain the percent monomer conversion data. The quenched mixture was then precipitated into 50 mL of cold methanol while stirring, filtered, washed with cold methanol to remove any unreacted monomer, and dried in a vacuum oven at RT overnight to a constant weight. Procedures for kinetic resolution of rac -DL by enantiomeric Y complexes ( R,R )- 4d and ( S,S )- 4d rac -DL was polymerized by ( R,R )- 4d or ( S,S )- 4d according to the above general procedure. The conversion of monomer was ~50% with the [ rac -DL]/[( R,R )- 4d ] molar ratio of 400 or 800 after 20 min, under which the conversion was 100% with rac - 4d as the catalyst. The polymerization was then quenched with benzoic acid/DCM (caution: avoid using nucleophiles such as methanol or acidified methanol as they react with the unreacted monomer, see Supplementary Figs. 30 , 31 ). The solvent was evaporated, and the solid residue was sublimated at 40–50 °C under vacuum to recover the pure unreacted monomer. The residue in the sublimator was dissolved in about 2 mL DCM, precipitated into 60 mL MeOH, filtrated, washed, and dried in vacuum to recover the polymer. The recovered unreacted monomer was analyzed by a chiral HPLC system to measure e.e . values, and the stereoselectivity factor s was calculated from Eq. ( 1) : 
    S = ln[ ( 1 - c)( 1 - ee_m)]/ln[ ( 1 - c)( 1 + ee_m)]
 (1) where \(c = 1 - \frac{{\left[ S \right] + \left[ R \right]}}{{\left[ S \right]_0 + \left[ R \right]_0}},\,ee_m = \frac{{\left[ S \right] - \left[ R \right]}}{{\left[ S \right] + \left[ R \right]}}.\) Polymer characterizations Measurements of polymer absolute weight-average molecular weight ( M w ), number-average molecular weight ( M n ), and molecular weight distributions or dispersity indices ( Đ = M w / M n ) were performed via gel-permeation chromatography (GPC). The GPC instrument consisted of an Agilent HPLC system equipped with one guard column and two PLgel 5 μm mixed-C gel permeation columns and coupled with a Wyatt DAWN HELEOS II multi (18)-angle light scattering detector and a Wyatt Optilab TrEX d RI detector; the analysis was performed at 40 °C using chloroform as the eluent at a flow rate of 1.0 mL min −1 , using Wyatt ASTRA 7.1.2 molecular weight characterization software (some presentative GPC traces are shown in Supplementary Figs. 61 – 66 ). 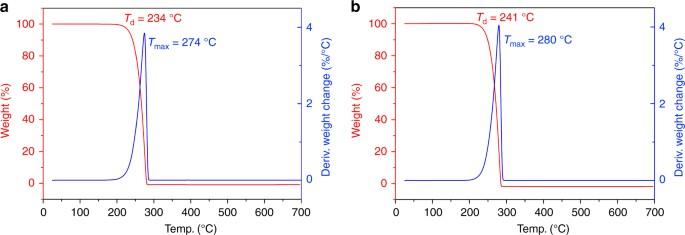Fig. 6 Thermal stability of P3HB derived from the ROP ofrac-DL.aTGA and DTG of P3HB produced by catalyst4a,Mn= 3.20 × 104g mol−1,Đ= 1.03, [mm] = 89%.bTGA and DTG of P3HB produced by catalyst4d,Mn= 1.19 × 105g mol−1,Đ= 1.03, [mm] > 99% The refractive index increment (d n /d c ) of P3HB was determined to be 0.0254 ± 0.0004 mL g −1 , obtained by batch experiments using Wyatt Optilab TrEX d RI detector and calculated using ASTRA software. Polymer solutions were prepared in chloroform and injected into d RI detector by Harvard Apparatus pump 11 at a flow rate of 0.25 mL min −1 . A series of known concentrations were injected and the change in refractive index was measured to obtain a plot of change in refractive index vs. change in concentration ranging from 0.4 to 4.0 mg mL −1 . The slope from a linear fitting of the data was the d n /d c of the polymer. The isolated low molecular weight samples were analyzed by MALDI-TOF MS; the experiment was performed on Microflex-LRF mass spectrometer (Bruker Daltonics, Billerica, MA) operated in positive ion, reflector mode using a Nd:YAG laser at 355 nm and 25 kV accelerating voltage. A thin layer of a 1% NaI solution was first deposited on the target plate, followed by 0.6 µL of both sample and matrix (dithranol in chloroform). External calibration was done using a peptide calibration mixture (4–6 peptides) on a spot adjacent to the sample. The raw data was processed in the FlexAnalysis software (version 3.4.7, Bruker Daltonics). T m and T g were measured by DSC on an Auto Q20, TA Instrument. All T m and T g values were obtained from a second scan after the thermal history was removed from the first scan. The second heating rate was 10 °C min −1 and cooling rate was 10 °C min −1 unless indicated otherwise in the polymerization tables. T d , defined by the temperature of 5% weight loss, and T max of the polymers were measured by TGA on a Q50 TGA Analyzer, TA Instrument. Polymer samples were heated from ambient temperatures to 700 °C at a heating rate of 10 °C min −1 . Values of T max were obtained from derivative (wt%/°C) vs. temperature (°C) plots, while T d and T onset values (initial and end temperatures) were obtained from wt% vs. temperature (°C) plots. 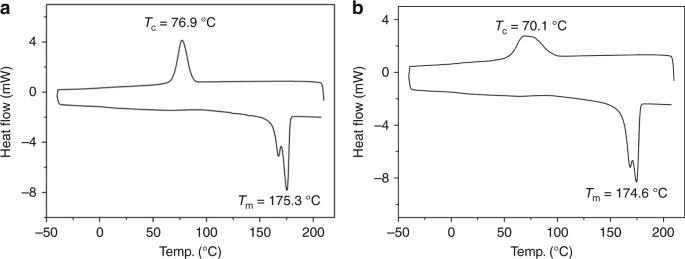Fig. 7 DSC curves of poly[(R)-3HB] materials.aProduced via chemical ROP ofrac-DL by (S,S)-[4d].bCommercial natural poly[(R)-3-hydroxybutyric acid] purchased from Sigma-Aldrich.TcandTmvalues taken from the cooling and second heating scans, respectively 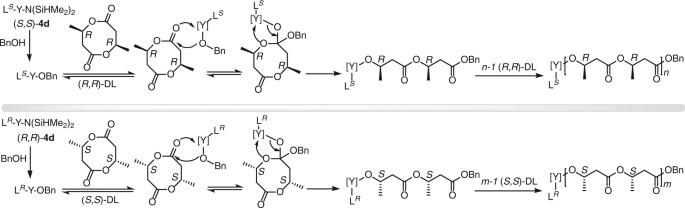Fig. 8 Proposed mechanism. Chemical scheme of the proposed catalyst-site controlled coordination-insertion mechanism for the ROP ofrac-DL byrac-4d Data availability The authors declare that the data supporting the findings of this study are provided in the main article and the Supplementary Information.